Printing three-dimensional tissue analogues with decellularized extracellular matrix bioink The ability to print and pattern all the components that make up a tissue (cells and matrix materials) in three dimensions to generate structures similar to tissues is an exciting prospect of bioprinting. However, the majority of the matrix materials used so far for bioprinting cannot represent the complexity of natural extracellular matrix (ECM) and thus are unable to reconstitute the intrinsic cellular morphologies and functions. Here, we develop a method for the bioprinting of cell-laden constructs with novel decellularized extracellular matrix (dECM) bioink capable of providing an optimized microenvironment conducive to the growth of three-dimensional structured tissue. We show the versatility and flexibility of the developed bioprinting process using tissue-specific dECM bioinks, including adipose, cartilage and heart tissues, capable of providing crucial cues for cells engraftment, survival and long-term function. We achieve high cell viability and functionality of the printed dECM structures using our bioprinting method. The ability to print tissue analogue structures through delivering living cells with appropriate material in a defined and organized manner, at the right location, in sufficient numbers, and within the right environment is critical for several emerging technologies. These technologies include, tissue-engineering scaffolds [1] , [2] , cell-based sensors [3] , drug/toxicity screening [4] and tissue or tumour models [5] . The concept of tissue or organ printing, often described as bioprinting [6] , is essentially an extension of the idea that uses additive manufacturing methods to build complex scaffold structures via a layer-by-layer process [7] , [8] , [9] , [10] . A crucial aspect of bioprinting is that the printing process must be cytocompatible, as it requires the dispensing of cell-containing media. This restriction reduces the choice of materials because of the necessity to operate in an aqueous or aqueous gel environment [11] , [12] . In extrusion-based printing, hydrogels that are solidified through either thermal processes or post-print cross-linking are being used for printing of cells to produce diverse tissues ranging from liver to bone using materials such as gelatin [13] , gelatin/chitosan [14] , gelatin/alginate [15] , gelatin/fibrinogen [16] , Lutrol F127/alginate [17] and alginate [18] . However, there are some concerns over the outcomes from these studies, such as the use of harsh cross-linking agents, like glutaraldehyde [14] . Elsewhere, osteogenic differentiation was not prominent on alginate gel and no differentiation was observed on Lutrol F127 (ref. 17 ). In addition, when alginate gel was used for printing of a cell-printed structure, only a minor fraction of cells in the construct could differentiate towards osteogenic lineage [17] . Normally, cells remain located specifically in their original deposited position during the whole culture period, as they are unable to adhere or degrade the surrounding alginate gel matrix [19] . This limited interaction between the cells within the gel can be explained by the noninteractive nature of alginate. Thus, although there were some successful reports about bioprinting of cell-printed structure, minimal cells–material interactions and inferior tissue formation are the foremost concerns. Actually, these materials cannot represent the complexity of natural extracellular matrices (ECMs) and thus are inadequate to recreate a microenvironment with cell–cell connections and three-dimensional (3D) cellular organization that are typical of living tissues. Consequently, the cells in those hydrogels cannot exhibit intrinsic morphologies and functions of living tissues in vivo . It is thus ideal if cells are provided the natural microenvironment similar to their parent tissue. Decellularized extracellular matrix (dECM) is the best choice for doing so, as no natural or man-made material can recapitulate all the features of natural extracellular matrix (ECM) [20] . Moreover, ECM of each tissue is unique in terms of composition and topology, which is generated through dynamic and reciprocal interactions between the resident cells and microenvironment [21] . Recent studies of cells and ECM isolated from tissues and organs highlight the necessity of tissue specificity for preserving selected cell functions and phenotype [20] , [22] , [23] , [24] , [25] . The dECM materials are harvested and typically processed as two-dimensional (2D) scaffolds from various tissues, including skin [26] , small intestinal submucosa [27] , where at the initial stages the infiltrating or seeded cell populations depend on diffusion of oxygen and nutrient for their survival until a supporting vascular network develops. However, printing tissue analogue structures requires a fabrication approach to devise a highly open porous 3D structure to allow the flow of nutrients [11] , [28] . Organ transplantation in an orthotopic location is considered as a definitive treatment for end-stage organ failure [23] , [24] , [29] . However, the demand for transplantable organs surpasses the number of available donor organs, compelling the manufacture of tissue or organs to address this unmet demand. Here we develop a bioprinting method for printing of cell-laden structure with novel dECM bioink capable of providing an optimized microenvironment conducive to the growth of 3D structured tissue, where the intrinsic cellular morphologies and functions can be reconstituted. We show the versatility and the functionality of our bioprinting process using various types of dECMs bioinks, including adipose, cartilage and heart tissues. As applications of these functional cell-printed constructs, we observe higher-order assembly of these cellular constructs with organized spatial patterns and tissue-specific gene expression. A key advantage of this methodology is the application of tissue-specific ECM, providing crucial cues for cells engraftment, survival and long-term function. Preparation of dECM bioink The method for printing of cell-laden construct using dECM bioink consists of a few steps ( Fig. 1 ). Decellularization of the ECM material is the initial step and practically, the goal is to maximize the removal of cellular material, while minimizing ECM loss and damage [30] . We successfully decellularized the adipose (adECM), cartilage (cdECM) and heart (hdECM) tissue after harvesting with a combination of physical, chemical and enzymatic process using slightly modified methods described elsewhere [31] , [32] , [33] . Furthermore, 0.1% peracetic acid solution in combination with 4% ethanol was used in the last step of the decellularization method, which is frequently considered as a disinfection step [34] . Efficiency of decellularization method was evaluated through DNA quantification assay and was found to be optimal for removing the cellular contents with ~98% reduction and only 39±15, 11±1 and 6.7±1.2 ng of DNA per mg of tissue remaining in the dECM of fat, cartilage and heart tissue, respectively ( Fig. 2 ). Hematoxylin and eosin (H&E) staining confirmed the absence of cells and cell debris in the matrix after decellularization ( Fig. 2b,c ) in all samples of dECMs, including those from the innermost regions of the processed tissues. Although the term decellularization has not been defined by quantitative metrics, <50 ng dsDNA per mg ECM dry weight and lack of visible nuclear material in H&E-stained tissue sections were reported to satisfy the objective of decellularization [30] . Thus, it can be said that we could effectively decellularize all the tissue samples. Regrettably, xenogeneic ECM obtained from pig and other animals may contain the Galα1,3Galβ1,4GlcNAc-R (Gal) epitope, which is a major factor in the hyperacute rejection of pig organ transplants in primates [35] . However, Gal epitope within porcine-derived ECM scaffold material was reported to elevate the serum antibody level, but no adverse reaction upon tissue remodelling was reported [35] . Thus, it is expected that dECMs used in this study will not elicit any inflammatory reaction upon implantation in a recipient. We also estimated the ECM components, like collagen (COL) and glycosaminoglycans (GAGs), before and after decellularization ( Fig. 2d–f ) with hydroxyproline assay and dimethylmethylene blue assay, respectively. The decellularization procedure adapted for heart tissue caused no noteworthy loss of COL and GAGs ( Fig. 2e ). In case of adipose tissue, the COL content increased slightly and the GAGs content reduced moderately after decellularization ( Fig. 2f ). As decellularization process removes all the cellular components along with lipids from the adipose tissue, COL contents seem to increase proportionately. For cartilage tissue, a significant loss of COL and GAGs were observed after decellularization ( Fig. 2d ). The reason behind variation of the proportion of ECM components was the difference of decellularization processes adapted in this study [30] . Cartilage has relatively denser ECM structure than that of heart, thus it requires more trypsinization and treatment with other enzymes, such as deoxyribonuclease (DNAse) and ribonuclease (RNAse), to remove all the cellular debris from ECMs. These enzyme treatments may be responsible for the reduction of COL and GAGs in decellularized cartilage tissue as trypsin treatment is known to cause partial removal of ECM constituents [30] . Unfortunately, the natural organization of structural fibres is lost by decellularization and reduction to a soluble powder and advantages can be gained when other proteins (not identified) were present in the extracts as shown by work of others [36] . We have evaluated the presence of proteins or peptides through sodium dodecyl sulphate (SDS)–PAGE ( Supplementary Fig. 1 ), which revealed the existence of various proteins within the dECMs used in this investigation and in accordance with other studies [37] . Thus, the presence of various proteins and peptides will ensure to gain the advantages by preparing cell-printed constructs using dECMs bioink. 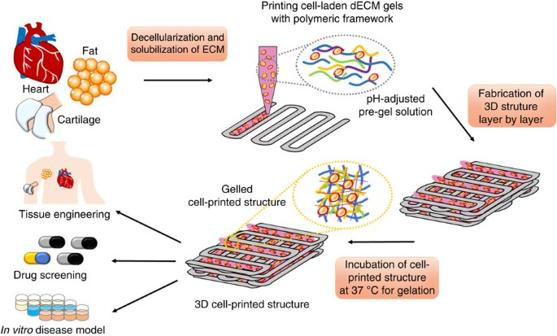Figure 1: Schematic elucidating the tissue printing process using dECM bioink. Respective tissues were decellularized after harvesting with a combination of physical, chemical and enzymatic processes, solubilized in acidic condition, and adjusted to physiological pH. Tissue printing was performed with the dECM bioink encapsulating living stem cells via a layer-by-layer approach followed by gelation at 37 °C. The 3D cell-printed structure has applications in various border areas including tissue engineering,in vitrodrug screening and tissue/cancer model. Figure 1: Schematic elucidating the tissue printing process using dECM bioink. Respective tissues were decellularized after harvesting with a combination of physical, chemical and enzymatic processes, solubilized in acidic condition, and adjusted to physiological pH. Tissue printing was performed with the dECM bioink encapsulating living stem cells via a layer-by-layer approach followed by gelation at 37 °C. The 3D cell-printed structure has applications in various border areas including tissue engineering, in vitro drug screening and tissue/cancer model. 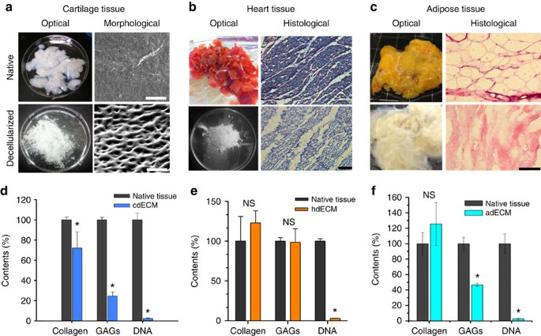Figure 2: Decellularization of the native tissues and their biochemical analysis. Optical and microscopic images of native and decellularized (a) cartilage tissue (scale bar, 50 μm), (b) heart tissue (scale bar, 100 μm), and (c) adipose tissue (scale bar, 100 μm). ECM components (Collagen and GAGs) and DNA contents of native and decellularized (d) cartilage (cdECM), (e) heart (hdECM) and (f) adipose (adECM) tissue. All experiments were performed in triplicate. Error bars represent s.d. (*P<0.05; NS, no significance). Full size image Figure 2: Decellularization of the native tissues and their biochemical analysis. Optical and microscopic images of native and decellularized ( a ) cartilage tissue (scale bar, 50 μm), ( b ) heart tissue (scale bar, 100 μm), and ( c ) adipose tissue (scale bar, 100 μm). ECM components (Collagen and GAGs) and DNA contents of native and decellularized ( d ) cartilage (cdECM), ( e ) heart (hdECM) and ( f ) adipose (adECM) tissue. All experiments were performed in triplicate. Error bars represent s.d. (* P <0.05; NS, no significance). Full size image Central to our approach is the development of dECM bioinks that can be extruded through the deposition nozzles in filamentary form, which then undergo gelation at physiological temperature and facilitates to retain the generated 3D structure. For translating dECM to 3D printing system, the dECM was solubilized to get a final concentration of 3%. However, the resulting solubilized dECM solution was acidic in nature and was adjusted to physiological pH prior to encapsulating cells while maintaining the temperature below 10 °C. The pH-adjusted dECM solution was designated as dECM pre-gel hereafter in this study, which behaved like a heat sensitive material that remains in the solution state at temperatures below 15 °C and transforms to gel when incubating at 37 °C for 30 min ( Fig. 3a ). 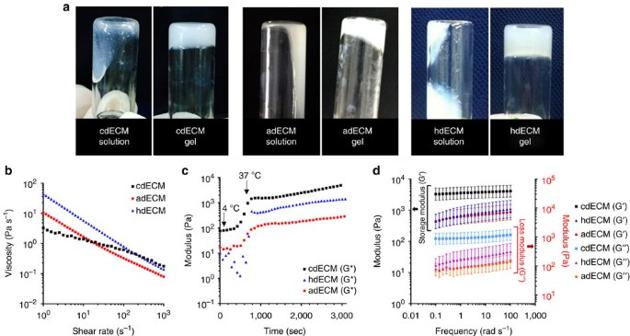Figure 3: Rheological behaviour of the dECM pre-gels. Sol to gel transition (a) of the dECM pre-gels prepared from cartilage dECM (cdECM), heart dECM (hdECM) and adipose dECM (adECM). Rheological properties of the dECM pre-gels (b) viscosity at 15 °C, (c) gelation kinetics from 4 °C to 37 °C. (Initial temperature: 4 °C, increment of 5 °C min−1with holding at 15 °C for 5 min, reaching to 37 °C, and maintaining 37 °C for 40 min), and (d) dynamic modulus at varying frequency at 37 °C. All experiments were performed in triplicate. Error bars represent s.d. Figure 3: Rheological behaviour of the dECM pre-gels. Sol to gel transition ( a ) of the dECM pre-gels prepared from cartilage dECM (cdECM), heart dECM (hdECM) and adipose dECM (adECM). Rheological properties of the dECM pre-gels ( b ) viscosity at 15 °C, ( c ) gelation kinetics from 4 °C to 37 °C. (Initial temperature: 4 °C, increment of 5 °C min −1 with holding at 15 °C for 5 min, reaching to 37 °C, and maintaining 37 °C for 40 min), and ( d ) dynamic modulus at varying frequency at 37 °C. All experiments were performed in triplicate. Error bars represent s.d. Full size image Characterization of dECM bioink Rheological properties of pH-adjusted dECM pre-gels were measured to evaluate their flow behaviour at temperatures below 15 °C to mimic the condition for printing. All dECM pre-gels showed shear thinning behaviour in the measured shear rate range ( Fig. 3b ). In the case of extrusion printing, one concern is the level of stress that cells endure during printing processes. We calculated the shear rate generated during the printing of dECM pre-gel and correlated it with the viscosity. The generated shear rate in our printing method through a 250 μm nozzle was determined in the range of 0.64–2.048 s –1 . The viscosities of the dECM solutions at 2 s −1 shear rate were 2.8 (for cdECM), 6.13 (for adECM) and 23.6 Pa s −1 (for hdECM) ( Fig. 3b ) when measured at 15 °C, which is similar to the other dECM gel reported in literature [38] . The storage and loss moduli of the dECM pre-gels were measured at 15 °C temperature that exhibited more like a liquid mater. However, when rheological properties were measured under oscillating condition after incubating the dECM pre-gels at 37 °C for 30 min, they behaved like a cross-linked gel and exhibited greater storage modulus than loss modulus ( Fig. 3d ). Thus, after gelation, the dECM gel can retain their shape and form, which is a prerequisite for fabrication of cell-printed constructs. In addition to the rheological properties, we also evaluated the gelation kinetics of the dECM pre-gels at varying temperatures starting from 4 to 37 °C with a temperature ramp of 5 °C and holding at 15 °C for 5 min. As Fig. 3c shows, the complex modulus started increasing soon after reaching the temperature beyond 15 °C and increased significantly as the temperature reached 37 °C. This observation indicates that dECM pre-gels started gelation immediately at temperature beyond 15 °C and formed a cross-linked gel at 37 °C within 30 min. Furthermore, it is interesting to note that although the viscosities of the three kinds of dECM pre-gels were similar; their storage moduli were different from each other. Pre-gel cdECM revealed quite larger storage modulus than those of the other two dECMs pre-gels (adECM and hdECM). The protein concentration of the final dECMs is an important determinant of their rheological properties as reported elsewhere [34] . Furthermore, the gelation characteristics of the dECM solutions are not simply COL chemistry but rather a result of the interplay of all of the components within the digested ECMs [34] . The method of decellularization also affects the rheological properties of final dECM solutions as the proportion of different components of the dECM were shown to vary depending upon the decellularization method adapted [30] . We have adapted different decellularization procedure through optimization for adipose, cartilage and heart tissue in this study, which possibly play a role in revealing dissimilar rheological properties of the obtained dECM solutions. Furthermore, the ratio and organization of various ECM components also dictate the mechanical properties of the native tissues like cartilage having a larger storage modulus than that of adipose or heart tissue. The native environment of tissue determines the cellular function and fate. Thus, we could assume that the cross-linked dECM gels from specific tissues will support their resident cells adequately. Cells in the adECM samples require a softer gel to mimic their natural environment for acquiring their inherent phenotype. On the other hand, chondrocytes require a favourable environment for obtaining their rounded shape with prominent curvature of the nucleus. Printing of cell-laden structure using dECM bioink The essential process to produce a functional tissue is a fabrication of dECM construct, allowing the encapsulating cells to migrate and connect to each other three dimensionally. We successfully produced 3D open porous structures of dECMs with polycaprolactone (PCL) framework using a multi-head tissue/organ building system (MtoBS) ( Fig. 4a and Supplementary Fig. 2 ) based on the 3D printing technique developed in house [39] . The MtoBS is capable of positioning one or more polymer or hydrogel or both at specific locations. We have applied different strategies for fabricating dissimilar tissue constructs. For heart tissue constructs, we have printed only the hdECM pre-gel without any synthetic polymer supporting framework ( Fig. 4a,b and Supplementary Fig. 2b ). On the other hand, we printed cartilage and adipose tissue construct by depositing the cell-laden dECM pre-gel following fabricating of PCL framework ( Fig. 4a,c,d ). However, we opted for two separate line width of the PCL framework, like 200 μm was chosen for cartilage tissue that needs more load-bearing support. For adipose tissue construct, we have selected finer line width, that is, 100 μm to reduce the stiffness. To elaborate the process of fabricating hybrid structure, we have first laid down a layer of PCL framework followed by the positioning of dECM pre-gel in every alternating gap between PCL lines to make the porous structure ( Fig. 4a , Supplementary Fig. 2 and Supplementary Movie 1 ). The process was repeated for every layer to produce the 3D construct. Thermal effect of PCL on cell viability has already been verified in the previous work and found to cause no/insignificant cell death [8] . One concern of printing constructs with the hybrid approach using PCL is that this would alter the overall cell environment, especially at the border of dECM-PCL. A few cells present at the boarder of dECM-PCL may experience the PCL environment, which is significantly stiffer than the cdECM [40] ; however, majority of the cell will experience the dECM surroundings as the cells were encapsulated within the dECM gel prior to printing. 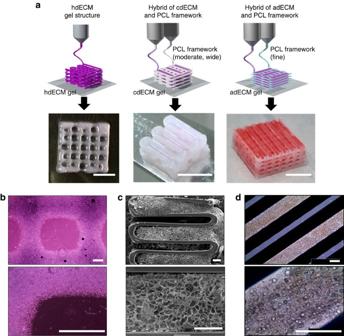Figure 4: Printing process of particular tissue constructs with dECM bioink. (a) Heart tissue construct was printed with only heart dECM (hdECM). Cartilage and adipose tissues were printed with cartilage dECM (cdECM) and adipose dECM (adECM), respectively, and in combination with PCL framework (scale bar, 5 mm). (b) Representative microscopic images of hdECM construct (scale bar, 400 μm), (c) s.e.m. images of hybrid structure of cdECM with PCL framework (scale bar, 400 μm) and (d) microscopic images of cell-printed structure of adECM with PCL framework (scale bar, 400 μm). Figure 4: Printing process of particular tissue constructs with dECM bioink. ( a ) Heart tissue construct was printed with only heart dECM (hdECM). Cartilage and adipose tissues were printed with cartilage dECM (cdECM) and adipose dECM (adECM), respectively, and in combination with PCL framework (scale bar, 5 mm). ( b ) Representative microscopic images of hdECM construct (scale bar, 400 μm), ( c ) s.e.m. images of hybrid structure of cdECM with PCL framework (scale bar, 400 μm) and ( d ) microscopic images of cell-printed structure of adECM with PCL framework (scale bar, 400 μm). Full size image We fabricated the desired 3D microperiodic structure by placing the cell-laden dECM pre-gel in between the PCL framework on a warm stage. The dECM pre-gel was maintained at temperatures below 15 °C during its extrusion from syringe. The cell-printed structure was gelled in a humidified incubator at 37 °C for 30 min. The printed gel remained stable on the deposited position throughout the culture period without separation for at least 14 days ( Fig. 5a–c and Supplementary Fig. 3 ). Furthermore, the system is capable of fabricating structures with various geometries needed for certain tissues. Using our bioprinting process, we successfully printed structures from 1 to 10 layers, as shown in Fig. 4a . Thus, it is not overwhelming to state that we can print constructs from thin to thick dimensions via proper positioning of this novel bioink encapsulating cells with engineered porosity for nutrient and oxygen supply depending on the requirements. We also observed the versatility of this method through printing two kinds of bioinks from different dECMs in a single construct ( Supplementary Movie 2 ), which could enable us to fabricate composite tissues. 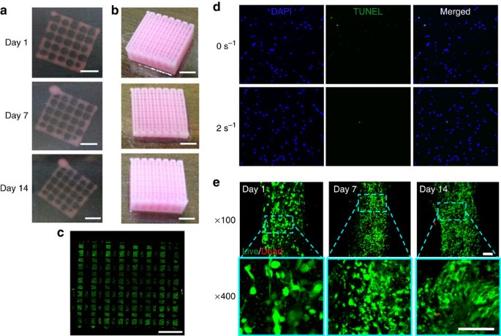Figure 5: Long-term stability and cellular compatibility of the printed tissue constructs. Representative images of the whole constructs prepared with hdECM (a) and adECM (b) at progressing days of cell culture (scale bar, 2 mm). Confocal image of the whole construct prepared with adECM at day 14 of culture (c) showing live cells (green dots) and dead cells (red dots) (scale bar, 2 mm). An image of the whole construct was reconstructed from ~32 images taken at different positions. Representative images of apoptosis through TUNEL (d) and Live/Dead (e) assays (scale bar, 100 μm). TUNEL assay displays very minimal apoptotic cells, which suggests that the generated stress at 2 s−1shear rate at the nozzle wall did not cause deleterious effect on the encapsulated cells and resulted similar apoptosis to the non-printed gel (0 s−1). Cell viability was >95% at day 1 and >90% at both day 7 and 14. Figure 5: Long-term stability and cellular compatibility of the printed tissue constructs. Representative images of the whole constructs prepared with hdECM ( a ) and adECM ( b ) at progressing days of cell culture (scale bar, 2 mm). Confocal image of the whole construct prepared with adECM at day 14 of culture ( c ) showing live cells (green dots) and dead cells (red dots) (scale bar, 2 mm). An image of the whole construct was reconstructed from ~32 images taken at different positions. Representative images of apoptosis through TUNEL ( d ) and Live/Dead ( e ) assays (scale bar, 100 μm). TUNEL assay displays very minimal apoptotic cells, which suggests that the generated stress at 2 s −1 shear rate at the nozzle wall did not cause deleterious effect on the encapsulated cells and resulted similar apoptosis to the non-printed gel (0 s −1 ). Cell viability was >95% at day 1 and >90% at both day 7 and 14. Full size image For printing of cell-laden dECM pre-gel, one important criterion is that the material should come out of the nozzle with minimum applied shear force. Otherwise, the applied shear force may cause damage to the cells and reduce the cell viability in the printed constructs [11] . We have checked the cell death that may take place by the generated shear stress through TUNEL assay that is capable of detecting the apoptotic cells. Shear rate of 2 s −1 was chosen to simulate the printing process. As it can be seen in Fig. 5d , there was very minimal cell death caused by the printing process and no difference in number of apoptotic cells were found in printed construct and the gel without printing. To obtain a desired cell number and cell distribution in the construct, higher cell viability of the printed construct should be maintained. The cell viability in the printed construct was found to be sufficiently high (>95%) when examined after 24 h ( Fig. 5e ). Cell-printed structure with only hdECM also revealed similar result of high viability of myoblasts after 24 h ( Supplementary Fig. 4 ). Actually, dECM gels possibly protect the cells through cushioning them during extrusion and allow cells to acquire the desired morphology during their residence in the gel. We also could observe the cell- to -cell connections in 3D within 24 h mimicking the in vivo conditions ( Fig. 5e ), which is very important for their survival and functions. Moreover, the dECM gels did not produce any deleterious effect on the cells or hindered their migration as the high cell viability (>90%) was maintained when the sample was examined on day 7 and 14 with active cell proliferation ( Fig. 5e ). Tissue-specific gene expression We investigated cellular morphologies and functions of the cell-laden constructs using stem cells, such as human adipose-derived stem cells (hASCs) and human inferior turbinate-tissue derived mesenchymal stromal cells (hTMSCs), a potential abundant cell source for clinical application from human inferior turbinate tissues generally discarded during turbinate surgery [41] , [42] . These cells have been shown to be promising for adipose tissue regeneration [25] and cartilage tissue regeneration [41] , respectively. To assess the differentiation of the printed stem cells, in particular encapsulating in dECM, tissue-specific gene expressions were analysed. Before demonstrating the superiority of each dECM material, cell proliferation test was conducted. This test verified that all the dECMs provide biocompatible microenvironment for cell proliferation and outperformed the other printable materials, such as COL and alginate ( Supplementary Figs 5 and 6 ). Among the various ECM components, COL was selected as a control for comparative analysis of target gene expression, because it is the most abundant component of ECM and has been used for cell printing [43] . Although, the major COL of cartilage is type II COL, not type I, we chose it as a control because of its increased application in cartilage tissue engineering. Direct differentiation of hTMSCs into chondrogenic lineage in cdECM was verified through qRT–PCR analysis. We normalized the target genes expressions with glyceraldehyde 3-phosphate dehydrogenase (GAPDH), as it shows least variation when cells were cultured on TCP over time ( Supplementary Fig. 7 ). On day 14, cells printed with cdECM revealed greater messenger RNA (mRNA) expressions of SOX9 that is an early chondrogenic transcription factor and type II COL than that of COL construct ( Fig. 6a ). Moreover, on day 3, SOX9, adhesion-related genes (focal adhesion kinase; protein tyrosine kinase 2) and integrin β1 were significantly greater than that of COL ( Supplementary Fig. 8 ), indicating the chondrogenic potential of cdECM constructs. Rat myoblast cells (L6, ATCC CRL-1458) were used to verify the effectiveness of hdECM for functional maturation of myoblasts. For assessment of the maturation level of myoblast in the hdECM structure, mRNA expression was analysed through qRT–PCR; in particular, the expression level of cardiac-specific genes like fast myosin heavy chain (Myh6) and alpha-sarcomeric actinin (Actn1). The hdECM constructs disclosed significantly higher levels of both the genes than that of the COL constructs during 14 days study period ( Fig. 6b ). Moreover, the expression of Myh6 and Actn1 were also higher in hdECM than that of COL at day 4 and 7 ( Supplementary Fig. 9 ), which signify the superiority of hdECM over COL gel. 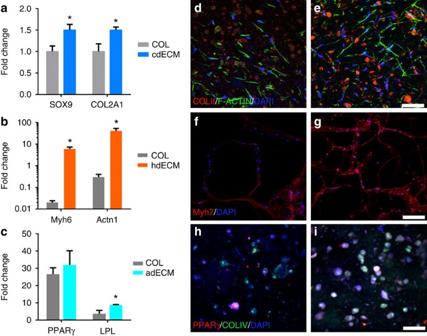Figure 6: Evaluation of differentiation into tissue-specific lineages and structural maturation of cells. Comparative gene expression analysis for (a) chondrogenic (SOX9 and COl2A1), (b) cardiogenic (Myh6 and Actn1) and (c) adipogenic (PPARγ and LPL) in COL and particular dECM (cdECM or hdECM or adECM) at day 14. Immunofluorescence images showing chondrogenic differentiation of hTMSCs in (d) COL and (e) cdECM constructs showing COL type II staining (COLII, red), cell nuclei (DAPI, blue) and F-actin (green) (scale bar, 50 μm). Structural maturation of myoblasts in (f) COL and (g) hdECM construct showing Myh7 (red) and cell nuclei (DAPI, blue) (scale bar, 200 μm). Adipogenic differentiation of hASCs in (h) COL and (i) adECM constructs showing PPARγ (red), COL IV (green) and cell nuclei (DAPI, blue) (scale bar, 50 μm). All experiments were performed in triplicate. Error bars represent s.d. (*P<0.05). Figure 6: Evaluation of differentiation into tissue-specific lineages and structural maturation of cells. Comparative gene expression analysis for ( a ) chondrogenic (SOX9 and COl2A1), ( b ) cardiogenic (Myh6 and Actn1) and ( c ) adipogenic (PPARγ and LPL) in COL and particular dECM (cdECM or hdECM or adECM) at day 14. Immunofluorescence images showing chondrogenic differentiation of hTMSCs in ( d ) COL and ( e ) cdECM constructs showing COL type II staining (COLII, red), cell nuclei (DAPI, blue) and F-actin (green) (scale bar, 50 μm). Structural maturation of myoblasts in ( f ) COL and ( g ) hdECM construct showing Myh7 (red) and cell nuclei (DAPI, blue) (scale bar, 200 μm). Adipogenic differentiation of hASCs in ( h ) COL and ( i ) adECM constructs showing PPARγ (red), COL IV (green) and cell nuclei (DAPI, blue) (scale bar, 50 μm). All experiments were performed in triplicate. Error bars represent s.d. (* P <0.05). Full size image Adipogenic differentiation has been shown to enhance under high-density conditions where the cells have a more rounded morphology and the cellular growth ceases [44] . As such, the high-density cell printing is an important step that will facilitate adipogenic differentiation for supporting adipogenesis in the culture groups. We have shown the possibility of printing cell-laden construct with high density (5 × 10 6 cells ml −1 ) using our bioprinting method without any deleterious effect on cell viability. Moreover, a significant increase in the expression of the master adipogenic regulators peroxisome proliferator-activated receptor gamma (PPARγ) and CCAAT/enhancer-binding protein alpha (C/EBPα) together with an increase in early adipogenic marker lipoprotein lipase (LPL) was observed when hASCs were cultured in adECM in comparison with COL and alginate ( Fig. 6c and Supplementary Fig. 10 ), widely used materials for cell printing [2] , [18] . The gene expression trends in the constructs showed increase in the expression of the adipogenic markers over time, consistent with a progression in differentiation, demonstrating the ‘adipoconductive’ nature of adECM. Thus, 3D printed constructs fabricated through our bioprinting method using dECM bioink supported differentiation and maturation of encapsulated cells and functionality of the respective tissues. Tissue formation Tissue formation was evaluated through immunohistological study. Supportive role of cdECM to differentiate hTMSCs into the chondrogenic lineage in cell-printed constructs with cdECM was verified through immunofluorescence imaging, which indicated that the cells synthesized type II COL within the construct ( Fig. 6d,e and Supplementary Fig. 11 ) and was in accordance with the mRNA expression results. We also verified the function of cdECM on enhancing cell adhesion by using F-actin staining ( Fig. 6e ). Most of the cells displayed spread morphology on the TCP ( Supplementary Fig. 12a ) and COL ( Supplementary Fig. 12b ); on the other hand, many cells were migrated into the depth of the cdECM ( Supplementary Fig. 12c ) and the cells were observed to be elongated and created mesh-like junctions in between them. This phenomenon corresponds to the expression of adhesion-related genes. It is also implied that cdECM have abundant residues to bind cells, which might have triggered the chondrogenesis transcription marker like SOX9 ( Supplementary Fig. 8 ). The maturation of myoblasts in cell-printed structure with hdECM was investigated by cardiac myosin heavy chain (β-MHC) staining and was compared with that of COL ( Fig. 6f,g and Supplementary Fig. 13 ), an abundantly available protein in the myocardium. The result showed that cells expressed higher level of β-MHC in the hdECM construct than that of COL and was also in accordance with the qRT–PCR result. In general, myoblasts were formed into the myofibres during the structural maturation. Subsequent to this, the differentiated myoblasts (myocytes) express the slow myosin heavy chain and synchronize with the native tissue. The slow myosin heavy chain is usually expressed in the newly formed cardiomyocytes. This phenomenon is associated with the graft survival; especially, the enhanced graft survival influences the alignment of the differentiated myoblasts in parallel with the host myocardial fibre [45] . The above finding advocates the potentiality of myoblasts printed hdECM structure for myocardial reconstruction. Upon differentiation of hASCs into the adipogenic lineage, they express PPARγ and COL IV. Cell-printed construct with adECM revealed substantial expression of PPARγ and COL IV ( Fig. 6h,i , and Supplementary Fig. 14 ) with higher level of fluorescence intensity to that of COL construct. These observations highlight the tissue-formation capabilities of our cell-printed constructs. In the present study, for the first time, tissue printing with particular dECM bioink that encompass either living hASCs or hTMSCs is demonstrated. Printed cell dECM constructs revealed higher levels of cell viability, differential lineage commitment and ECM formation. This study addresses recent advancement in the field of bioprinting for engineering biological tissues, consisting of cells encapsulated in dECM with specific organization and matrix composition. The adapted printing technology of depositing cell-laden dECM hydrogel that we used can fulfil several important requirements of tissue-engineered grafts, including tissue-specific matrix materials, engineered interconnected porosity, the introduction of pertinent cells, and the opportunity to explore organizational aspects in tissue regeneration. Encapsulation of cells within dECM hydrogel prior to the deposition process facilitates the formation of cell-laden, viable printed constructs [17] . In this way, the cell loading can be altered and different types of cells can be laid down in tissue-mimicking architectures. We have also shown that our printing method does not cause stress-induced apoptosis of the encapsulated cells and high level of cell viability was achieved. Moreover, being a robust dispensing method, our bioprinting technique can produce constructs of anatomically relevant (centimetre scale) sizes for tissue replacement. Pepsin digestion cleaves the telopeptide regions of the COL, which allows solubilization of the dECM in dilute acids [43] . We could achieve highly concentrated dECM solution with adequate viscosity for printing of cell-laden constructs. When pH values of these dECM solutions were adjusted, they behaved similar to temperature-sensitive pre-gel materials, allowing printing of well-defined 3D constructs that were transformed into physically cross-linked gel at 37 °C. The structures were stable in vitro without the need for chemical cross-linking. We used dECMs processed from tissues, such as adipose, cartilage and heart, for printing of particular tissue analogue. Likewise, this method can also be extended to ECM from other tissues with little modification. At present, tissue-engineering strategies utilizing ECM materials are being successfully used clinically for the regeneration of a range of tissues [46] , [47] . The main advantage of utilizing ECM material is that it facilitates constructive remodelling at the implantation site and encourages specific tissue formation rather than forming inferior and less functional scar tissue [36] . We demonstrated that human living progenitor cells survive the generated shear stress during the printing process of cell-laden dECM hydrogel with a high level of cell survival, which is in line with previous reports [17] . This can be explained through the shear thinning behaviour of ECM hydrogel, which results in a decrease in shear stress. This phenomenon of shear thinning is a common behaviour for polymeric gel or hydrogel and has been described in detail elsewhere [48] . We could print a precisely defined but flexible designed structure with a homogenous distribution of cells within the construct. In addition, to improve the mechanical integrity of the printed dECM hydrogel constructs, cell-laden hydrogels were combined with structurally stiffer synthetic polymers, such as PCL for cartilage construct. The versatility of of our bioprinting method was demonstrated through printing two different bioinks from various dECMs in a single constructs. The capability to print different dECM hydrogels simultaneously exemplified the ability of our process to reproducibly print heterogeneous 3D structures comprising various kinds of dECM. As a follow-up step, we demonstrated the printing of heterogeneous constructs (that is, printed with different kinds of dECM at different locations). However, further studies should be directed to investigate the heterogeneous tissue formation based on this approach. The ECM microenvironment plays a fundamental role in directing and mediating the differentiation of stem cell while culturing them [49] . There is strong evidence supporting that this instruction conveyed through both receptor ligand interactions, as well as mechanical signalling events, which in turn stimulate the important signal transduction pathways and control the cellular function [49] . The cell–ECM interactions are extremely complex in nature and justify the need for a tissue-specific approach while creating the native stem cell niche. Recent studies have validated this tissue-specific outlook and shown the manifestation of enhanced functions [20] and intricate tissue formation [22] , [23] when site-specific ECM scaffolds were being employed. The ECM scaffolds were shown to have the capacity to direct tissue-specific stem cell lineage commitment and maintaining the phenotype of mature cell populations [50] . Here, we obtain a synergistic effect through combining the beneficial effects of dECM with tissue printing process to get a cell-laden construct with engineered porosity in a tissue-specific manner. With this approach, we were able to generate a tissue analogue in vitro with either adipogenic or chondrogenic potential. In particular, we demonstrated that hASCs or hTMSCs could be printed via encapsulating in dECM pre-gel and that the in vitro culture did not modify cell survival and proliferation, but increased the commitment of stem cells towards either adipogenic lineage within dECM from fat tissue or chondrogenic lineage within cartilage dECM. Enhanced structural maturation of myoblasts was observed in constructs prepared with dECM from heart tissue. ECM has been shown to guide tissue morphogenesis through modulating cell–cell interactions [51] , [52] . Thus, we demonstrated that tissue printing with dECM bioink is an attractive option that opens up new avenues for both in vitro and in vivo tissue reconstruction. Nevertheless, there are other potential application areas where a tissue analogue structure developed by our bioprinting method is worthwhile ( Fig. 1 ). In vitro models of human physiology and pathology can be developed using our bioprinting method and can benefit to convincingly and accurately predict the outcomes of in vivo drug administrations and potential toxic exposures, if any [4] . Furthermore, cancer model can be developed by recreating the microenvironmental characteristics representative of tumours in vivo with our bioprinting method with dECM that provide cancer tissue-mimicking 3D environment [5] . Materials As synthetic biomaterial, FDA-approved PCL (molecular weight=70,000–90,000 g mol −1 ; Polyscience, Inc., PA, USA) was used. SDS solution 10% and 1M Tris-HCL solution were purchased from Bioneer, South Korea. Triton X-100 was purchased from Affymetrix-USB, Santa Clara, CA. Pepsin, DNAse and RNAse A were purchased from Sigma-Aldrich, St Louis, MO. Sodium chloride (NaCl) was purchased from Junsei, Japan. Unless otherwise stated, cell culture reagents were obtained from Sigma-Aldrich. Decellularization of tissues Porcine cartilage and heart from a 6-month-old pig was collected from a nearby slaughter house and used with approval from the supplier. The left ventricle was isolated from the whole porcine heart. Heart tissue decellularization was conducted by following the protocol published elsewhere with slight modification [32] . Tissues were cut into pieces of about 1 mm in thickness. The chopped heart tissue was stirred in 1% SDS in phosphate-buffered saline (PBS) solution for 48 h followed by treatment with 1% Triton X-100 solution for 30 min. The decellularized heart tissue was washed using PBS at least for 3 days. The hyaline cartilage was collected from porcine articular cartilage and decellularized by following the protocol published elsewhere with modification [33] . Briefly, the minced cartilage was placed into a hypotonic Tris-HCL buffer solution (10 mM Tris–HCL, pH 8.0) and 6 cycles of freezing (at −80 °C) and thawing (at 37 °C) were conducted. The cartilage slurry was homogenized and treated with 0.25% trypsin in PBS for 24 h at 37 °C with vigorous agitation. The trypsin solution was replaced with the fresh one at every 4 h. Trypsinized cartilage slurry was washed with a hypertonic buffer solution (1.5 M NaCl in 50 mM Tris-HCL, pH 7.6) and treated with nuclease solution (50 U ml −1 DNAse and 1 U ml −1 RNAse A in 10 mM Tris–HCL, pH 7.5) with gentle agitation at 37 °C for 4 h. To remove all the enzymes, the enzyme-treated cartilage slurry was washed with the hypotonic Tris–HCL solution for 20 h following treatment with 1% Triton X-100 solution for 24 h. The decellularized cartilage tissue was washed at least for 3 days to remove all the detergent. The adipose tissue was collected from hospital (St Mary’s Hospital, Seoul, South Korea) after liposuction of seven different female donors at the ages between 35 and 54 with informed consent and under approval from the Catholic University of Korea Institutional Review Board. The collected tissue was centrifuged to separate the oil and blood from the tissue. The adipose tissue was washed with PBS solution and decellularized with 0.5% SDS solution for 48 h with changing the solution every 12 h. Decellularized adipose tissue was then treated with isopropanol to remove the lipid for 48 h with changing the isopropanol every 12 h followed by washing several times with PBS solution. Finally, all the decellularized and delipidated tissues were treated with a solution of 0.1% peracetic acid in 4% ethanol for 4 h followed by washing several times with PBS solution and distilled water. The obtained dECMs from heart, cartilage and adipose tissues were lyophilized and stored in −20 °C freezer. Biochemical characterization of dECMs To verify the extent of decellularization, the residual DNA was measured and histological sections were analysed with H&E staining. ECM components like COL and GAGs in the decellularized tissue were also assessed. For DNA quantification, all the dECMs were digested in 1 ml of papain solution (125 μg ml −1 papain in 0.1 M sodium phosphate with 5 mM Na 2 -EDTA and 5 mM cysteine-HCl at pH 6.5) for 16 h at 60 °C. Papain solution without sample for using as a diluent in biochemical assays was also incubated. Native tissues of similar weight were also digested in a same manner as controls. The DNA content was determined using Hoechst 33258 assay [53] . The fluorescence intensity was measured to assess the amount of remaining DNA within the dECMs and the native tissue using a fluorescence spectrophotometer (TECAN, Switzerland; excitation wavelength: 360 nm, emission wavelength: 450 nm). The standard curve for DNA was generated in advance using calf thymus DNA and used for quantifying the DNA in samples. For histological evaluation, both native and decellularized tissues were fixed in 4% formalin, washed several times with distilled water, embedded in OCT compound, sectioned using a cryotome (Leica CM1850 Cryostat, Germany), stained with H&E, and observed under microscope. The GAGs content was estimated via quantifying the amount of sulphated glycosaminoglycans using 1,9-dimethylmethylene blue solution [54] . The absorbance was measured with microplate reader at wavelength of 492 nm. The standard curve was made using chondroitin sulphate A in advance and used for estimating the sulphated glycosaminoglycans in samples. The total COL content was determined via a conventional hydroxyproline assay [55] . The absorbance of the samples was measured at 550 nm and quantified by referring to a standard curve made in advance with hydroxyproline. Preparation of dECM solution and pre-gel Lyophilized dECM was crushed into powder using a mortar and pestle with the help of liquid N 2 . Required amount of dECM powder was weighed and digested in a solution of 0.5 M acetic acid with 10 mg of pepsin for 100 mg dECM (P7125, Sigma-Aldrich) for 48 h. After complete solubilization of dECM, the solution was centrifuged (only for adipose dECM) to remove the particulate things if any and used for further examinations. The pH of dECM solution was in the range of 2.8–3. The pH was adjusted with dropwise addition of cold 10 M NaOH solution while maintaining the temperature below 10 °C to avoid gelation of the dECM. The pH-adjusted dECM pre-gel was stored in refrigerator at 4 °C. Rheological characterization Rheological investigations were conducted on an Advanced Rheometric Expansion System (TA Instrument, USA) using 25 mm diameter plate geometry. To assess the viscosity, steady shear sweep analysis of various dECM pre-gels were performed at a constant temperature of 15 °C. Dynamic frequency sweep analysis was conducted to measure the frequency-dependent storage (G′) and loss (G″) moduli of various dECM gels in the range of 1–1,000 rad s –1 at 2% strain after incubation for 30 min at 37 °C. A temperature sweep was used to study the gelation kinetics of dECM pre-gels. The complex modulus was measured at each temperature while the dECM pre-gels were subjected to a temperature ramp in the range of 4–37 °C with a increment rate of 5 °C min −1 . In addition, at 15 °C, the dECM pre-gels were held for 5 min. All measurements were conducted in triplicate. Cell encapsulation in the dECM pre-gel hASCs and hTMSCs were used for assessment of the effectiveness of adECM and cdECM on adipogenic and chondrogenic differentiation of adult stem cells, respectively. The cells were isolated and cultured by a previously described method [41] , [42] , [56] . Rat myoblast cells (L6, ATCC CRL-1458) were used for verifying functional enhancement of myoblasts in the hdECM. hASCs and L6 cells were cultured in the DMEM high glucose supplemented with 10% fetal bovine serum and 1% antibiotics (penicillin/streptomycin), and hTMSCs were cultured in the αMEM supplemented with 10% fetal bovine serum and 1% antibiotics (penicillin/streptomycin). All the cells used were from passage 2 to 5. Cultured cells were detached from the tissue culture plate with 0.25% trypsin solution, centrifuged at 1,500 r.p.m. for 3 min, suspended in fresh media and counted. To maintain the same osmotic pressure, 10 × concentrated culture media was added to the pH-adjusted dECM pre-gel (1/10 th volume) and the suspended cells were mixed thoroughly with the pH-adjusted ECM pre-gel. The concentration of cells used was from 1 to 5 × 10 6 cells ml −1 . All processes were conducted on ice. The prepared bioink was loaded in a sterilized syringe for cell printing. Printing of cell-laden construct A MtoBS, a bioprinting system developed in our lab, with six different syringe holders and capable of simultaneously dispensing six different materials, was used for printing of cell-laden construct. PCL was loaded in a syringe and heated to 80 °C to melt the polymer. The dECM pre-gel encapsulated cells were loaded to the other syringe and maintained at temperatures below 15 °C. Cell-printed constructs were fabricated according to the method described elsewhere [39] . We used two syringes for constructing each structure, one containing PCL and maintained at 80 °C, the other one loaded with cell-laden pre-gel and maintained at temperatures below 15 °C. The applied pneumatic pressure was in the range of 400–650 kPa for fabrication of the PCL framework. The cell-laden pre-gel was dispensed using a plunger-based low-dosage dispensing system. In the process of printing synthetic polymer, temperature of the molten PCL comes down very fast in the air gap before reaching the stage. Cell viability and apoptosis test Cells were under a relatively high shear-stressed environment when the mechanical perturbations were applied to the cells by dispensing bioinks. Therefore, we verified the viability and apoptosis of cells after the printing. For cell apoptosis assay, we selected hdECM as a representative bioink due to its highest viscosity among the developed bioinks. The hTMSCs were encapsulated at a concentration of 5 × 10 5 cells ml −1 into 3% hdECM pre-gel and the prepared bioink was loaded into the piston syringe. The grid type structure of 100 μm in thickness was fabricated with the hdECM bioink at 2 s −1 shear rate, which was selected to simulate the shear rate generated during printing. Finally, the fabricated structure was cross-linked by incubating at 37 °C temperature for 30 min. After 24 h of incubation in the complete medium, the structure was fixed by 4% paraformaldehyde and treated with the DeadEnd Fluorometric TUNEL System kit (Promega, WI) following manufacturer’s protocol with little modification. We treated all reagents for a longer time than that of the time mentioned in the protocol due to the larger thickness of the structure. The TUNEL system can measure the fragmented DNA of apoptotic cells by catalytically binding fluorescein-12-dUTP; thus, the fluorescein-12-dUTP-labelled DNA in the fabricated structure was visualized by confocal microscope (Olympus FluoView FV1000, Tokyo, Japan). Cell nucleus was counterstained by DAPI (GBI Labs, WA). To conduct viability test, cell-printed structures with dECM was evaluated by staining with live and dead assay kit (LIVE/DEAD Cell Viability Assays, Invitrogen Life Technologies, USA) following manufacturer’s protocol. Gene expression analysis through RT–PCR After culturing the constructs for the specified time period, total RNA of cells was isolated using TRIzol reagent (Invitrogen Life Technologies, USA) following the manufacturer’s protocol. RNA concentration was measured using a Nanodrop (Thermo Scientific, USA). Reverse transcription was performed with the cDNA synthesis kit (Thermo Scientific, USA) following manufacturer’s instructions. Gene expression was analysed quantitatively with SYBR-green using 7500 Real-Time PCR system (Applied Biosystems, Life Technologies, USA). The primers and probes for collagen type II (COL2A1), SOX9, protein tyrosine kinase 2, Integrin β1, PPARγ, C/EBPα, LPL, Myh6, Actn1, beta-actin, 18S ribosomal RNA and GAPDH were designed on the basis of published gene sequences (NCBI and PubMed). We checked the expression patterns of various endogenous control genes (GAPDH, beta-actin and 18S ribosomal RNA) of cells cultured on TCP over time. GAPDH has shown low level of variance among samples over time than the other genes ( Supplementary Fig. 7 ). Thus, we have chosen GAPDH as an endogenous control for our study. Expression levels for each gene were normalized with GAPDH and analysed using the 2 −ΔΔCT method. Each sample was assessed in triplicate. Immunohistological study The cell-printed structure was harvested and fixed with a solution of 4% paraformaldehyde after 14 days culture. The structure was embedded in OCT compound and sectioned using cryotome in 10-μm thickness. The sliced samples were washed repeatedly with PBS solution to remove OCT compound and then permeabilized with a solution of 0.1% Triton X-100 in PBS for 5 min. To reduce non-specific background, sections were treated with 0.2% bovine serum albumin solution in PBS for 20 min. For visualization of differentiation and maturation of stromal cells to chondrogenic cells, sections were immunostained using primary antibody against anti-collagen II antibody (1:100; Abcam, UK) followed by incubation with Alexa Fluor 594 goat anti-mouse antibody (1:100; Invitrogen, CA). Sections were also stained with phalloidin-FITC solution (1:100; Sigma-Aldrich, MA) for 40 min and DAPI for 15 min. The adipogenic cell-printed structure was harvested and fixed with a solution of 4% paraformaldehyde after 14 days culture and stained following similar protocol using PPARγ (1:100; Santa Cruz Biotechnology Inc, Catalogue No. sc-81152) and Collagen IV (1:100; Santa Cruz Biotechnology Inc, COL4A5 (H-234): sc-11360). Secondary antibody of Alexa Fluor 594 goat anti-mouse antibody (1:100; Invitrogen, CA) and Alexa Fluor 488 goat anti-rabbit antibody (1:100; Invitrogen, CA) were used and counterstained with DAPI. For detection of the myotube formation in the hdECM construct, sections were stained with anti-heavy chain cardiac myosin antibody (1:100; Abcam), followed by incubation with secondary goat anti-mouse-Alexa 594 antibody (1:100) and counterstained with DAPI. For F-actin expression analysis, the cells were seeded on the each material (tissue culture plate, TCP; COL and cdECM gel), and were cultured for 3 days and stained with phalloidin-FITC solution for 40 min and DAPI for 15 min. Stained samples were visualized and images were captured using a confocal microscope. Statistical analysis All data are expressed as mean±s.d. All statistical analysis was performed by using SigmaPlot software (ver. 10.0, Systat Software Inc., San Jose, CA). Statistical significance was determined by a one-way analysis of variance. Differences were considered to be statistically significant at P <0.05. How to cite this article : Pati, F. et al . Printing three-dimensional tissue analogues with decellularized extracellular matrix bioink. Nat. Commun. 5:3935 doi: 10.1038/ncomms4935 (2014).